The induction and function of the anti-inflammatory fate of TH17 cells 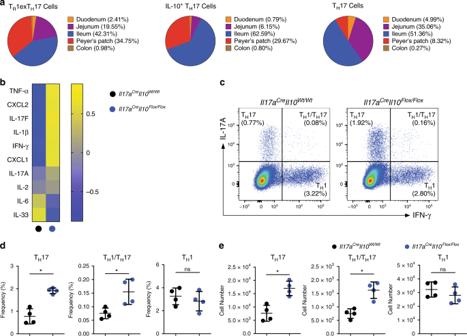Fig. 1: TH17 derived IL-10 contributes to intestinal homeostasis. aTissue distribution of the indicated cell populations within the intestine. Cells were isolated from indicated intestinal tracts of the Fate+mice. All cell populations are pre-gated on Foxp3−, YFP+, CD4+T cells and then described as TR1exTH17(IL-10eGFP+IL17AKata−), IL-10+TH17 (IL-10eGFP+IL17AKata+) and TH17 (IL-10eGFP–IL17AKata+) cells on the basis of the reporter molecules. Cell numbers from three cumulative experiments are used to calculate mean percentage values of the indicated cell populations in different intestinal compartments.bHeatmap showing normalized mRNA expression value (Z-score) of different cytokines/chemokines in small intestinal tissues.c. Flow cytometric analysis of small intestinal CD4+T cells isolated from the indicated mouse lines under steady state. Intracellular staining for both IL-17A and IFN-γ was then performed to identify TH17 (IL-17A+IFN-γ−), TH1/TH17 (IL-17A+IFN-γ+) and TH1 (IL-17A−IFN-γ+) cells. A pre-gate on CD4+T cells is applied.d,eStatistical analysis of frequencies (d) and numbers (e) are reported. One representative experiment out of three is shown. Each dot represents one mouse (nwild type= 4,nKO= 4). Mean ± S.D.; ns, not significant; *P< 0.05 by Mann–WhitneyUtest. Source data are provided as a Sourcedatafile. T H 17 cells exemplify environmental immune adaptation: they can acquire both a pathogenic and an anti-inflammatory fate. However, it is not known whether the anti-inflammatory fate is merely a vestigial trait, or whether it serves to preserve the integrity of the host tissues. Here we show that the capacity of T H 17 cells to acquire an anti-inflammatory fate is necessary to sustain immunological tolerance, yet it impairs immune protection against S . aureus . Additionally, we find that TGF-β signalling via Smad3/Smad4 is sufficient for the expression of the anti-inflammatory cytokine, IL-10, in T H 17 cells. Our data thus indicate a key function of T H 17 cell plasticity in maintaining immune homeostasis, and dissect the molecular mechanisms explaining the functional flexibility of T H 17 cells with regard to environmental changes. The consequences of dysfunctional immune adaptation are clear: the immune cells either fail to mount a protective response to lethal infections, or they overreact to non-harmful antigens and in doing so, induce disparate immune mediated inflammatory diseases (IMIDs). It is therefore both fundamentally and clinically relevant to reveal the molecular mechanisms underlying this phenomenon of immune adaptation. T H 17 cells—a subset of CD4 + T cells—exemplify immune adaptation. On the one hand, T H 17 cells can have a full effector function protecting the host from pathogens with the associated risk of developing IMIDs [1] , [2] , [3] , [4] , [5] . On the other hand, T H 17 cells can also acquire an anti-inflammatory fate characterized by secretion of the anti-inflammatory cytokine, IL-10 [6] , [7] , [8] . However, the relevance of this T H 17 anti-inflammatory fate and the consequences of its impairment have not yet been fully explored. T H 17 cells are abundant in the intestine [6] , but it remains to be tested whether by acquiring an anti-inflammatory fate, they contribute to intestinal immune homeostasis by blocking the development of a pathological response and preserving the tissue integrity. Furthermore, whether this anti-inflammatory fate negatively impacts T H 17 mediated immunity to pathogens is also unknown. Finally, the exact molecular mechanism behind this cellular adaptation also remains to be clarified. Even though the key molecular pathways for the differentiation of CD4 + T cells into T H 17 cells have been studied extensively [9] , [10] , [11] , [12] , investigation into the mechanisms that promote the anti-inflammatory fate of mature T H 17 cells has just begun [7] , [13] , [14] , [15] , [16] . On the basis of in vitro screenings, we proposed that TGF-β controls the expression of IL-10 in CD4 + T cells during their in vitro differentiation into T H 17 cells [7] , [17] . However, whether TGF-β also plays a key role in vivo and on already matured T H 17 cells, and through which molecular signalling, remain to be studied. It is known that upon engagement of TGF-β with TGFBR1/R2 on CD4 + T cells, TGFBR2 trans phosphorylates TGFBR1, which propagates signalling by phosphorylating Smad2 and Smad3. Once Smad2 and Smad3 form a heteromeric complex with the common mediator Smad4, they translocate to the nucleus to trans-activate several genes. It has been shown that while Smad2 promotes RORγt activity (i.e. the key transcriptional factor of T H 17 cell differentiation), Smad3 impairs it [18] , [19] . Furthermore, Smad4 and SKI protein bind together and repress the Rorγt promoter, thus when Smad4 gene is deleted from CD4 + T cells, IL-6 can induce T H 17 cells without TGF-β [2] . Interestingly, in embryonic stem cells, Smad2 and Smad3 complex cannot access the target genes without TIF1-γ [20] . Therefore, TIF1-γ is considered an alternative pathway to Smad4. Indeed, Smad2/Smad3-TIF1-γ complex controls the differentiation of hematopoietic stem/progenitor cells in response to TGF-β, while Smad2/3-Smad4 complex regulates the proliferation of those cells [21] . Recent data suggest that the deletion of Tif1g in CD4 + T cells decreases the expression of IL-17A and increases IL-10 while the cells are differentiating into T H 17 cells [22] . Of note, this latter study is performed either in vitro or it addresses the role of TIF1-γ during the differentiation of CD4 + T cells into T H 17 cells, rather than in vivo or on mature T H 17 cells. Therefore, the role of TGF-β on mature T H 17 cells and through which pathways TGF-β signals, are still unclear. In this study, we find that the anti-inflammatory fate of T H 17 cells contributes to maintaining intestinal immune homeostasis. In addition, our data show that the anti-inflammatory fate of T H 17 cells impairs an effective immune response to S . aureus , but is essential to control the resolution of the intestinal inflammation. Furthermore, we show that all this is orchestrated by TGF-β via Smad3 and Smad4 signalling and not via TIF1-γ. Finally, we extended part of these findings to human biology. Together, these observations broaden our understanding about how late fate decision of T H 17 cells is controlled and about the physiological implications behind T H 17 plasticity. T H 17 derived IL-10 contributes to intestinal homeostasis We previously showed that some T H 17 cells can express IL-10 (IL-10 + T H 17) and eventually fully convert into bona fide T R 1 cells (T R 1 exTH17 ): the anti-inflammatory fate of T H 17 cells [6] , [7] . Of note, the identity of these T R 1 exTH17 cells has been previously shown at both the transcriptional and functional levels [7] . However, the spatial distribution of these different cell statuses (i.e. IL-10 + T H 17 and T R 1 exTH17 cells) remained to be defined. We used the Fate + ( Il17a Cre / Katushka , Rosa26 - STOP Flox / Flox YFP ( R26 YFP ), Il10 eGFP , Foxp3 RFP ) mice and assessed the presence of T H 17 (Foxp3 RFP− IL-17A Katushka+ IL-10 eGFP− R26 YFP+ ), IL-10 + T H 17 cells (Foxp3 RFP− IL-17A Katushka+ IL-10 eGFP+ R26 YFP+ ) and T R 1 exTH17 cells (Foxp3 RFP− IL-17A Katushka − IL-10 eGFP+ R26 YFP+ ) in lymphoid and in intestinal tissues. We observed that the majority of these two T H 17-derived IL-10 producing cell populations (i.e. IL-10 + T H 17 cells and T R 1 exTH17 cells) reside in the Peyer’s Patches (PP) and in the ileum (Fig. 1a ). Considering that the small intestine and PP host several other types of anti-inflammatory cells, such as Foxp3 + Treg and T R 1 cells, which also secrete high levels of IL-10 [23] , [24] , [25] , we wondered whether the anti-inflammatory fate of T H 17 cells is redundant for the intestinal homeostasis. To this end, we crossed Il17a Cre mice with Il10 Flox / Flox and R26 YFP mice (from here on referred to as Il17a Cre Il10 Flox / Flox ) (Supplementary Fig. 1a ). First, we confirmed the efficiency of IL-10 deletion in T H 17 cells in vivo and in vitro (Supplementary Fig. 1b–e ). Then we investigated whether intestinal homeostasis in these mice was altered. Although we did not observe any obvious intestinal tissue damage microscopically (Supplementary Fig. 1f ), many pro-inflammatory genes such as Il1b , Il17f , Cxcl1 , Ifng and Tnfa are elevated in the intestinal tissues of Il17a Cre Il10 Flox / Flox mice, compared to their littermate control mice ( Il17a Cre Il10 Wt / Wt ) under steady state conditions (Fig. 1b ). Furthermore, a more detailed cellular analysis revealed that under steady state conditions, there was an accumulation of T H 17 and T H 1/T H 17 cells in the small intestine of the Il17a Cre Il10 Flox / Flox mice compared to their wild-type littermate controls. Of note, the T H 1 cell population was comparable in frequency and number between the Il17a Cre Il10 Flox / Flox and control mice, suggesting that T H 17 cell derived IL-10 has a specific capacity to regulate T H 17 cell expansion in the intestine (Fig. 1c–e ). Fig. 1: T H 17 derived IL-10 contributes to intestinal homeostasis. a Tissue distribution of the indicated cell populations within the intestine. Cells were isolated from indicated intestinal tracts of the Fate + mice. All cell populations are pre-gated on Foxp3 − , YFP + , CD4 + T cells and then described as T R 1 exTH17 (IL-10 eGFP+ IL17A Kata− ), IL-10 + T H 17 (IL-10 eGFP+ IL17A Kata+ ) and T H 17 (IL-10 eGFP– IL17A Kata+ ) cells on the basis of the reporter molecules. Cell numbers from three cumulative experiments are used to calculate mean percentage values of the indicated cell populations in different intestinal compartments. b Heatmap showing normalized mRNA expression value (Z-score) of different cytokines/chemokines in small intestinal tissues. c . Flow cytometric analysis of small intestinal CD4 + T cells isolated from the indicated mouse lines under steady state. Intracellular staining for both IL-17A and IFN-γ was then performed to identify T H 17 (IL-17A + IFN-γ − ), T H 1/T H 17 (IL-17A + IFN-γ + ) and T H 1 (IL-17A − IFN-γ + ) cells. A pre-gate on CD4 + T cells is applied. d , e Statistical analysis of frequencies ( d ) and numbers ( e ) are reported. One representative experiment out of three is shown. Each dot represents one mouse ( n wild type = 4, n KO = 4). Mean ± S.D. ; ns, not significant; * P < 0.05 by Mann–Whitney U test. Source data are provided as a Source data file. Full size image Next, we profiled the IL-10 expression in different types of immune cells to assess the different potential contribution to the phenotype observed in the Il17a Cre Il10 Flox / Flox mice. We observed that more than 90% of the cells that co-express IL-10 and YFP (indicating IL-17A production) in the small intestine are CD4 + T cells (Supplementary Fig. 1g ). Finally, we tested whether Il17a Cre Il10 Flox / Flox mice acquired an extra intestinal spontaneous immune dysregulation, but we could not observe any immune abnormality in the thymus, spleen and other peripheral lymphoid organs (Supplementary Fig. 2 ). These data reveal the distribution of the IL-10 + T H 17 cells and T R 1 exTH17 cells along the small intestinal tract. Moreover, these data suggest that the anti-inflammatory fate of T H 17 cells plays a non-redundant role in maintaining the cellular and molecular immune homeostasis in the small intestine. IL-10 deletion in T H 17 enhances antibacterial immunity We next hypothesized that IL-10 deletion in IL-17A producing cells may lead to more efficient immunity at the expense of immunological tolerance. To test this hypothesis, we first used a S. aureus infection mouse model and then an intestinal inflammation mouse model followed by a spontaneous resolution phase. We and others have previously shown that intravenous infection of S. aureus promotes the accumulation and activation of IL-10-producing T H 17 cells at the intestinal barrier [6] , [7] , [26] . Mechanistically we showed that the superantigen of S. aureus , staphylococcus aureus enterotoxin B (SEB), induces a cytokine storm and rapid induction/expansion of intestinal T H 17 cells [6] . Here we first immunized the Il17a Cre Il10 Flox / Flox mice with heat killed S. aureus and then infected them to test the efficiency of bacterial clearance (Fig. 2a ). We observed that the Il17a Cre Il10 Flox / Flox mice had a lower bacterial burden compared to control mice ( Il17a Cre Il10 Wt / Wt ) in the spleen, small intestine and the liver (Fig. 2b ). We also confirmed the frequency and the number of both T H 17 and T H 1/T H 17 in Il17a Cre Il10 Flox / Flox mice were increased after treatment, as already observed under steady state conditions (Fig. 2c–e ). These results suggest that IL-10 deletion in IL-17A producing cells leads to a more efficient immune response against S . aureus . Fig. 2: IL-10 deletion in T H 17 enhances antibacterial immunity. T H 17 derived IL-10 impairs the development of an efficient immunity against S. aureus . a A schematic depiction of the experimental plan. b Colony-forming units (CFUs) of S. aureus from different organs. Data are cumulative of two independent experiments. Each dot represents one mouse ( n wild type = 7, n KO = 7). Mean ± SEM. ; * P < 0.05 by Mann–Whitney U test. c Flow cytometric analysis of small intestinal CD4 + T cells after S. aureus infection. Small intestinal lymphocytes were isolated from the indicated mouse lines and intracellular staining for both IL-17A and IFN-γ was performed to identify T H 17 (IL-17A + IFN-γ − ), T H 1/T H 17 (IL-17A + IFN-γ + ) and T H 1 (IL-17A − IFN-γ + ) cells. A pre-gate on CD4 + T cell is applied. One representative experiment out of three is shown. d , e Statistical analysis of frequencies ( d ) as well as numbers ( e ) are reported. One representative experiment out of three is shown. Each dot represents one mouse ( n wild type = 5, n KO = 5). Mean ± S.D. ; ns, not significant; * P < 0.05 by Mann–Whitney U test. Source data are provided as a Source data file. Full size image IL-10 deletion in T H 17 impairs intestinal immune regulation Next, we tested whether IL-17A-producing cell derived IL-10 plays an essential role during the resolution of inflammation in the small intestine. Thus, we challenged mice with anti-CD3 monoclonal antibody (mAb) treatment, a mouse model that we and others have previously established to induce a transient inflammation in the small intestine followed by the re-establishment of immunological tolerance [6] , [7] , [25] , [27] , [28] . We found that Il17a Cre Il10 Flox / Flox mice were more susceptible to inflammation induced weight loss compared to control mice ( Il17a Cre Il10 Wt / Wt ) (Fig. 3a ). Furthermore, the small intestines of the Il17a Cre Il10 Flox / Flox mice showed more severe tissue damage, represented by disrupted villi structures and edema compared to control mice (Fig. 3b ). In addition, we observed a selective accumulation of T H 17 cells and T H 17/T H 1 cells in the intestine of the Il17a Cre Il10 Flox / Flox mice (Fig. 3c–e ). We next questioned whether a different expression of IL-10R among the T H 17, T H 17/T H 1 and T H 1 cells could justify the selective accumulation of T H 17 cells and T H 17/ T H 1 but not of T H 1 cells in the Il17a Cre Il10 Flox / Flox mice. In line with what we published previously [25] , we indeed observed that T H 17 and T H 17/T H 1 cells express higher levels of IL-10R compared to T H 1 cells (Supplementary Fig. 3a, b ). Fig. 3: IL-10 deletion in T H 17 impairs intestinal immune regulation. a Percentage of initial body weight after anti-CD3 mAb. The arrows indicate the injection of anti-CD3 mAb. Data are cumulative of three independent experiments. Mean ± SEM. ; * P < 0.05, by two-way ANOVA with Bonferroni’s post test. b Representative histological pictures of H&E stained small intestines after anti-CD3 mAb treatment. For the statistical analysis on the right, one representative experiment out of two is shown. Each dot represents one mouse ( n wild type = 3, n KO = 3). Mean ± S.D. ; * P < 0.05 by Welch’s t -test. c Flow cytometric analysis of small intestinal CD4 + T cells after anti-CD3 mAb treatment. Small intestinal lymphocytes were isolated from the indicated mouse lines and intracellular staining for both IL-17A and IFN-γ was performed to identify T H 17 (IL-17A + IFN-γ − ), T H 1/T H 17 (IL-17A + IFN-γ + ) and T H 1 (IL-17A − IFN-γ + ) cells. A pre-gate on CD4 + cell is applied. d , e Statistical analysis of frequencies ( d ) and numbers ( e ) are shown. One representative experiment out of three is shown. Each dot represents one mouse ( n wild type = 5, n KO = 5). Mean ± S.D. ; ns, not significant; ** P < 0.01 by Mann–Whitney U test. Source data are provided as a Source data file. Full size image Collectively, these data indicate that the lack of IL-10 expression in IL-17A producing cells promotes immunity against S . aureus infection, but leads to impaired resolution of the immune response. TGF-βRII is required for mature T H 17 cells to produce IL-10 Despite the fact that the molecular signals inducing IL-10 in naïve CD4 + T cells have been largely explored, the molecular mechanisms that control IL-10 production in mature T H 17 cells in vivo remain unknown. TGF-β is an obvious candidate considering its effect on naive CD4 + T cells. To this end, we first differentiated T H 17 cells in vitro, FACS sorted IL-17A producing CD4 + T cells and then re-stimulated these cells in the presence of increasing doses of TGF-β. These results confirmed our previous findings [7] and further showed that TGF-β promotes IL-10 production also in mature T H 17 cells in a concentration-dependent manner (Supplementary Fig. 4a–d ). However, this was an in vitro experiment and whether this is also the case in vivo remained to be tested. Therefore, we tested the role of TGF-β on mature T H 17 cells using a loss-of-function approach. To this end, we crossed Tgfbr2 Flox / Flox with the Fate + mice (Supplementary Fig. 5a ). This newly generated Tgfbr2 Flox / Flox Fate + mouse model allowed us to specifically and selectively delete Tgfbr2 gene in IL-17A-producing cells, and in the meantime to track the T H 17 cell fate as well as cytokine profile. We first confirmed that the deletion of Tgfbr2 occurs in a T H 17-specific manner in Tgfbr2 Flox / Flox Fate + (Supplementary Fig. 5b ). Next, we tested whether Tgfbr2 -deficient T H 17 cells have any impairment in up-regulating IL-10 expression when cultured in vitro. We found that both the IL-10 + T H 17 population and T R 1 exTH17 population were reduced in cultured CD4 + T cells isolated from Tgfbr2 Flox / Flox Fate + mice compared to CD4 + T cells isolated from littermate controls (Fig. 4a, b ). Of note, we didn’t observe an obvious defect of primary T H 17 cell differentiation with Tgfbr2 Flox / Flox Fate + cells (Supplementary Fig. 5c, d ), which is in line with the previous observation that IL-17A Cre -mediated gene deletion did not affect primary T H 17 cell proliferation and differentiation [29] . Fig. 4: TGF-βRII is required for mature T H 17 cells to produce IL-10. a Flow cytometric analysis of in vitro cultured total CD4 + T cells. Cells were polarized under T H 17 condition for 5 days. A pre-gate on viable (DAPI − ), CD4 + T cell population is applied. b Statistical analysis of IL-10 + T H 17 and T R 1 exTH17 cells is shown by one representative experiment out of three. Each dot represents one mouse ( n wild type = 3, n KO = 5). Mean ± S.D. ; * P < 0.05, *** P < 0.001 by Welch’s t -test. c Flow cytometric analysis of small intestinal CD4 + T cells after anti-CD3 mAb treatment. The indicated reporter mouse lines were used. 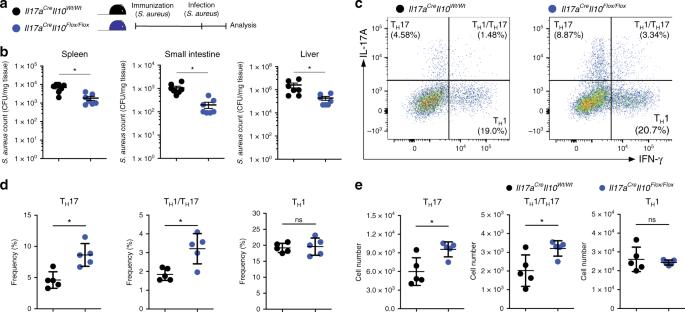Fig. 2: IL-10 deletion in TH17 enhances antibacterial immunity. TH17 derived IL-10 impairs the development of an efficient immunity againstS. aureus.aA schematic depiction of the experimental plan.bColony-forming units (CFUs) ofS. aureusfrom different organs. Data are cumulative of two independent experiments. Each dot represents one mouse (nwild type= 7,nKO= 7). Mean ± SEM.; *P< 0.05 by Mann–WhitneyUtest.cFlow cytometric analysis of small intestinal CD4+T cells afterS. aureusinfection. Small intestinal lymphocytes were isolated from the indicated mouse lines and intracellular staining for both IL-17A and IFN-γ was performed to identify TH17 (IL-17A+IFN-γ−), TH1/TH17 (IL-17A+IFN-γ+) and TH1 (IL-17A−IFN-γ+) cells. A pre-gate on CD4+T cell is applied. One representative experiment out of three is shown.d,eStatistical analysis of frequencies (d) as well as numbers (e) are reported. One representative experiment out of three is shown. Each dot represents one mouse (nwild type= 5,nKO= 5). Mean ± S.D.; ns, not significant; *P< 0.05 by Mann–WhitneyUtest. Source data are provided as a Source data file. Top panels are pre-gated on Foxp3 − CD4 + T cells. Bottom panels are gated on YFP + cells, as shown, and the indicated populations are identified on the basis of the reporter molecules as follows: T R 1 exTH17 cells: IL-10 eGFP+ IL-17a Kata− ; IL-10 + T H 17 cells: IL-10 eGFP+ IL-17a Kata+ ; T H 17 cells: IL-10 eGFP– IL-17a Kata+ . d , e Frequencies ( d ) and numbers ( e ) of the indicated populations are shown. One representative experiment out of three is shown. Each dot represents one mouse ( n wild type = 5, n KO = 5). Mean ± S.D. ; ns, not significant; * P < 0.05, ** P < 0.01 by Mann–Whitney U test. f . Experimental design for Co-transfer of total CD4 + T cells isolated from wild-type Fate + mouse and Tgfbr2 Flox/Flox Fate + mouse lines. g . Flow cytometric analysis of small intestinal co-transferred CD4 + T cells after anti-CD3 mAb treatment. Small intestinal lymphocytes were isolated from the indicated mouse lines and intracellular staining was then performed to identify the indicated cell populations in combination with reporter molecules for IL-10 (eGFP) and IL-17a lineage (YFP). All cell populations are pre-gated on CD4 + T cells. h Frequencies of T R 1 exTH17 and IL-10 + T H 17 in G is shown by one representative experiment out of two. Each dot represents one recipient mouse ( n = 3). Mean ± S.D. ; * P < 0.05, *** P < 0.001 by Welch’s t -test. Source data are provided as a Source data file. Full size image Finally, we examined whether T H 17 cells require TGF-βRII in order to produce IL-10 in vivo. We observed that under steady state conditions, intestinal CD4 + T cells marked by YFP (indicating Tgfbr2 deletion) from Tgfbr2 Flox / Flox Fate + mice had an obvious impairment in IL-10 and IL-17A production compared to those cells isolated from Tgfbr2 Wt / Wt Fate + mice (Supplementary Fig. 5e–g ). Since TGF-β promotes the expression of Foxp3, as a control we tested whether the small expression of Foxp3 + among the intestinal R26 YFP+ CD4 + T cells was dysregulated in the Tgfbr2 Flox/Flox Fate + mice. However, we did not observe any statistically significant dysregulation of Foxp3 and more importantly no difference in the number of Foxp3 + YFP + cells between the Tgfbr2 Flox/Flox Fate + and Tgfbr2 Wt / Wt Fate + mice (Supplementary Fig. 5h, i ). We then injected anti-CD3 mAb to induce a transient intestinal inflammation in the small intestine of these mice. Similar to what we observed by using the Il17a Cre Il10 Flox / Flox mice, Tgfbr2 Flox / Flox Fate + were more susceptible to intestinal inflammation compared to the relative control. The Tgfbr2 Flox/Flox Fate + lost more weight and had a more severe intestinal pathology than control Tgfbr2 Wt / Wt Fate + mice (Supplementary Fig. 6a, b ). We then harvested the intestinal tissues and analysed the lymphocyte composition. We observed that both the frequency and the amount of IL-10 + T H 17 cells and T R 1 exTH17 cells from the intestines of Tgfbr2 Flox / Flox Fate + mice were significantly lower than those from WT Fate + mice (Fig. 4c–e ). Of note, similar to what is seen under steady state conditions, we did not observe statistically significant changes in the expression of Foxp3 among R26 YFP+ CD4 + T, nor did we observe differences in the number of Foxp3 + R26 YFP+ cells between the Tgfbr2 Flox/Flox Fate + and Tgfbr2 Wt / Wt Fate + mice (Supplementary Fig. 6c, d ). To exclude the possibility that reduced IL-10 production from the CD4 + YFP + cells of Tgfbr2 Flox / Flox Fate + mice was a consequence of more severe inflammation, we co-transferred CD4 + T cells from both CD45.2 Tgfbr2 Flox / Flox Fate + mice and CD45.1/2 Tgfbr2 Wt / Wt Fate + mice into Rag1 −/− mice. After we engrafted the cells, we injected anti-CD3 mAb and finally harvested the cells. We found that even when the cells resided in the same environment, Tgfbr2 -deficient T H 17 cells lost their ability to express IL-10 compared to wild-type cells, which still produced IL-10 (Fig. 4f–h ). We also observed that Tgfbr2 -deficient R26 YFP+ T H 17 cells expanded and failed to preserve the expression of IL-17A (Supplementary Fig. 6e ), suggesting a role of TGF-β signalling in controlling proliferation and IL-17A maintenance in this particular experimental setting. Taken together, these data indicate that mature T H 17 cells intrinsically require signalling via TGF-βRII to promote the expression of IL-10 in vitro and in vivo. TGF-β signals via Smad3/4 to regulate IL-10 in T H 17 cells The next step was to explore the signalling pathway that drives IL-10 expression upon TGF-β engagement with its receptor on mature T H 17 cells. After TGF-β engages its receptor, Smad2 and Smad3 complex is phosphorylated and by binding to either TIF1-γ or Smad4, translocates into the nucleus to activate gene expression [21] . Whether either Smad4 or TIF1-γ controls TGF-β-mediated IL-10 expression in mature T H 17 cells remained to be tested. We first examined the role of TIF1-γ in the expression of IL-10 in T H 17 cells. To this end, we made Tif1g Flox / Flox Fate + mice, which similar to the Tgfbr2 Flox / Flox Fate + mice described above, in order to specifically deplete Tif1g in Il17a producing cells (Supplementary Fig. 7a ). After inducing intestinal inflammation in these mice, we observed that both IL-10 + T H 17 cells and T R 1 exTH17 cells remain comparable between Tif1g Flox / Flox Fate + mice and their wild-type littermate controls, suggesting that TIF1-γ is not required for IL-10 production in T H 17 cells in vivo (Supplementary Fig. 7b–d ). We then evaluated whether Smad4 is important for TGF-β-mediated IL-10 expression. To address this, we first created Smad4 Flox / Flox Fate + mice in order to delete Smad4 in T H 17 cells (Supplementary Fig. 8a ). Smad4 -deficient CD4 + T cells had a slight, but significant impairment in IL-10 production when cultured under T H 17 conditions in vitro (Supplementary Fig. 8b, c ). These mice were then injected with anti-CD3 mAb and IL-10 + T H 17 and T R 1 exTH17 cell populations were analysed. In line with the in vitro observations, both types of cells were reduced in the small intestines of Smad4 Flox / Flox Fate + mice compared with the wild-type control mice (Fig. 5a–c ). Fig. 5: TGF-β signals via Smad3/4 to regulate IL-10 in T H 17 cells. a Flow cytometric analysis of small intestinal CD4 + T cells after anti-CD3 mAb. The indicated reporter mouse lines were used. Top panels are pre-gated on Foxp3 − , CD4 + T cells. Bottom panels are pre-gated on YFP + cells, and the indicated populations are identified on the basis of the reporter molecules as follows: T R 1 exTH17 cells: IL-10 eGFP+ IL-17a Kata− ; IL-10 + T H 17 cells: IL-10 eGFP+ IL-17a Kata+ ; T H 17 cells: IL-10 eGFP− IL-17a Kata+ . b , c Frequencies ( b ) and numbers ( c ) of T R 1 exTH17 , IL-10 + T H 17 and T H 17 cells in A are one representative experiment out of three. Each dot represents one mouse ( n wild type = 5, n KO = 5). Mean ± S.D. ; ns, not significant; * P < 0.05, ** P < 0.01 by Mann-–Whitney U test. d Experimental design of knocking out Smad3 in in vitro differentiated mature T H 17 cells by using CRISPR/Cas9 technology. e Flow cytometric analysis of in vitro cultured mature T H 17 cells after knocking out Smad3 by using gRNAs targeting Smad3. Cells were pre-gated on viable CD4 + T cells. NT, non-targeting control. Each dot represents an individual gRNA ( n NT = 2, n Smad3 = 3). Mean ± S.D. ; ** P < 0.01 by Welch’s t -test. Source data are provided as a Source data file. Full size image Finally, we also determined the role of Smad3 in regulating IL-10 production in T H 17 cells. We disrupted the function of Smad3 by using either Crispr/Cas9 mediated gene depletion (Fig. 5d, e ), or small chemical inhibitor SIS3 in in vitro differentiated T H 17 cells (Supplementary Fig. 9a, b ). In both cases, we observed that the induction of IL-10 in in vitro differentiated T H 17 cells by TGF-β was impaired when Smad3 was deleted/blocked. These data suggest that Smad3 is also required for TGF-β induced IL-10 production in T H 17 cells in vitro. Taken together, these data show that while TIF1-γ is dispensable, Smad4 and Smad3 are necessary for TGF-β mediated IL-10 induction in mature T H 17 cells. Smad3 and Smad4 activate Il10 transcription in T H 17 cells We next sought to test whether Smad3 and Smad4 bind to the Il10 promoter in mature T H 17 cells. First, we tested whether phospho-Smad3 translocates into the nucleus shortly after TGF-β stimulation. Nuclear extracts of T H 17 cells were immunoblotted and we observed phospho-Smad3 in the nuclei of these cells (Fig. 6a ). Next, we tested whether Smad3 and Smad4 are able to induce Il10 gene transcription. We first cloned Il10 proximal promoter (−1444 to +1) in the pGL2 vector upstream of Luciferase reporter gene, and Smad3 and Smad4 genes in pCMV and pCMVβ mammalian expression vectors respectively. Co-transfection of Il10 proximal promoter with increasing concentrations of either only Smad3 or only Smad4 expression plasmids did not result in significant upregulation of luciferase activity. However, when increasing concentrations of Smad4 plasmid were co-transfected with a constant amount of Smad3 plasmid, a significant increase in Il10 -luciferase activity was observed (Fig. 6b ). These data suggest that Smad3 and Smad4 synergistically activate the Il10 promoter. Fig. 6: Smad3 and Smad4 activate Il10 transcription in T H 17 cells. a Western blot of T H 17 cell-total/nuclear extracts challenged with or without TGF-β for 30 min. One representative experiment out of two is shown. b Schematic representation of the proximal murine Il10 promoter (from −1444 to +1 bp) driving the expression of the luciferase reporter gene ( luc ). The predicted binding sites for Smad3 and Smad4 as well as the Il10 TSS are depicted (top). Relative Luc activity driven by Smad3 and Smad4 on proximal Il10 promoter (bottom). Mean ± SEM ( n = 3). * P < 0.05, ** P < 0.01, and *** P < 0.001 by ordinary two-way ANOVA and Tukey’s multiple comparisons test. c Schematic representation of the proximal murine Il10 promoter (from −1444 to +1 bp) indicating the predicted binding sites for Smad3 and Smad4 and the depicted amplicons A (from −416 to −278 bp), B (from −929 to −756 bp), and C (from −365 to −171 bp) (top) that were used to amplify the chromatin Immunoprecipitated DNA. Smad3 and Smad4 Chromatin immunoprecipitation (ChIP) of sorted T H 17 cells challenged with or without TGF-β (bottom). One representative experiment out of three is shown. d Proximity Ligation Assay (PLA) using sorted T H 17 cells challenged with or without TGF-β. White arrows indicate positive Smad3/Smad4 interaction signal (red dots) superimposed on nuclei stained with DAPI (blue). Scale bar represents 10 μm. Number of PLA spots per cell and the number of PLA positive cells are reported in the box. One representative experiment out of two is shown. *** P < 0.001 for comparison by χ 2 test. Source data are provided as a Source d ata file. Full size image In order to show that Smad3 and Smad4 directly bind the Il10 promoter in mature T H 17 cells, we performed Chromatin Immunoprecipitation (ChIP) experiments with FACS sorted T H 17 cells stimulated with or without TGF-β for 30 min. We found that 30 min after TGF-β treatment, both Smad3 and Smad4 accessed and bound the Il10 promoter on the −929/−756 element. Of note, between −929/−756 and −286/−283 base pairs on Il10 promoter lie predicted Smad3/4 binding sites (Fig. 6c ). As a negative control, we interrogated the GAPDH TATA box promoter region where Smad3 and Smad4 proteins do not bind, and as expected we did not see any signal. Finally, in order to show that Smad3 and Smad4 proteins form a complex in T H 17 cells, we performed Proximity Ligation Assay (PLA) in FACS sorted T H 17 challenged for 30 min with TGF-β, using a plus and a minus ligation probe specific for anti-mouse Smad3 and anti-rabbit Smad4 antibodies, respectively. Confocal microscopic images reveal that the Smad3/4 complexes are only visible in the nucleus of T H 17 cells challenged with TGF-β (Fig. 6d ). Interestingly, this protein complex forms 3–5 bright, closely spaced foci per cell. The PLA spots were located in the rim of the T H 17 cell nucleus associated with the nuclear membrane. Taken together, these results show that Smad3 and Smad4 proteins are instructed by TGF-β signal, form a nuclear complex that bind to the proximal Il10 promoter and transactivates Il10 transcription in T H 17 cells. TGF-β promotes IL-10 expression in human T H 17 cells We tested whether human T H 17 cells isolated from the intestine can also produce IL-10. We observed that a small but consistent frequency of CD4 + T cells isolated from healthy colon tissues from 14 human donors, co-produce IL-17A and IL-10 (Fig. 7a ). Next, we wondered whether human T H 17 cells can also acquire the expression of IL-10 when stimulated with TGF-β. We therefore isolated circulating CD45RA low CD25 − IL-17A + (T H 17) cells from human blood using the IL-17A secretion assay and cultured the isolated T H 17 cells in the presence of increasing TGF-β concentrations. The purity of the T H 17 cells isolated from human blood was always more than 95% (for a representative purity plot see Supplementary Fig. 10a ). Upon examining the CD4 + Foxp3 − T cell compartment (see Supplementary Fig. 10b for the gating strategy), we observed that approximately half of the sorted cells, that were formerly IL-17A + , ceased to produce IL-17A (i.e. they become exT H 17 cells) while the other half retained IL-17A expression. However, this phenomenon was not affected by TGF-β (Fig. 7b ). In contrast, TGF-β promoted IL-10 expression in both T H 17 cells and exT H 17 cells in a concentration-dependent manner (Fig. 7b ). Finally, increasing TGF-β concentrations appeared to slightly reduce the frequency and the numbers of IL17A + IFN-γ + and IFN-γ + producing cells (Supplementary Fig. 10c, d ). Furthermore, increasing the TGF-β concentrations did not have a reproducible effect on Foxp3 expression in human peripheral blood-isolated T H 17 cells (Supplementary Fig. 10e ). Collectively, these results show that human T H 17 cells from the intestine and from peripheral blood, are able to produce IL-10 and furthermore, that TGF-β is able to promote dose dependent IL-10 expression in human peripheral blood derived T H 17 cells. Fig. 7: TGF-β promotes IL-10 expression in human T H 17 cells. a Two representative dot plots of CD4 + T cells extracted from healthy human colonic tissue, stained intracellularly for IL-17A and IL-10. The diagrams show the frequencies of IL-17A + /IL-10 + within the T H 17 cells (left) and within the total CD4 + T cell (right) ( n = 14) b Representative dot plots of T H 17 cells isolated from human blood donor, stimulated and cultured under increasing TGF-β1 concentrations for 5 days and finally stained for IL-17A and IL-10 intracellularly. The graphs below show the percentages of IL-17A + /IL-10 − , IL-17A + /IL-10 + and IL-17A − /IL-10 + cells from four different blood donors. P values were calculated between the lowest TGF-β and highest TGF-β concentration conditions by Mann–Whitney U test ( n = 4). Source data are provided as a Source data file. Full size image T H 17 cells are usually found in the inflamed tissues of IMID patients such as the central nervous system, the kidney, the joints and the heart. However, they are also abundant in the small intestine of healthy individuals without causing any overt diseases [30] , [31] , [32] . The T H 17 cell plastic behaviour allowing them to acquire both pro- and anti-inflammatory fate can explain such ubiquitous presence and consequences: pathological or physiological. Our data show that it is in fact mainly in the ileum and Peyer’s patches of mice where these cells acquire their anti-inflammatory fate. This suggests that continuous plasticity from T H 17 cells to IL-10 producing T H 17 cells and possibly to T R 1 exTH17 cells impairs the pathogenic immune reaction of effector T H 17 cells in the intestinal tract. Supporting this, when T H 17 cell-derived IL-10 is lacking, the cellular and molecular immune homeostasis of the intestine is disturbed, showing the relevance of the anti-inflammatory fate of these cells. This effect is remarkable considering that only a relatively small fraction of T H 17 cells acquire an anti-inflammatory function. Finally, our data show that also human T H 17 cells acquire the regulatory phenotype when exposed to TGF-β1. Despite the above, we did not observe macroscopic tissue damage in the Il17a Cre Il10 Flox/Flox mice. One explanation is the compensatory mechanism which could be exerted by the presence of other regulatory T cells, such as Foxp3 + Treg cells and T R 1 cells able to produce IL-10 [23] , [25] . Indeed, it has to be considered that only a fraction of T R 1 cells originate from the T H 17 cells, while the rest originate from other cells, including probably T H 1 cells [33] . Thus, the latter T R 1 cell fraction is still functional in this mouse model. Another explanation is the composition of the intestinal microbiota of our mice. It is possible that under different specific pathogen free conditions, also Il17a Cre Il10 Flox/Flox mice develop microscopically evident intestinal inflammation. Interestingly, we observed a specific expansion of intestinal T H 17 and T H 1/T H 17 cells, but not of T H 1 cells in our Il17a Cre Il10 Flox/Flox mouse model. One possible explanation of this cell-selective control mediated by IL-10 is that both T H 17 and T H 1/ T H 17 cells express higher level of IL-10R compared to T H 1 cells. Alternatively, one could consider that this is due to a dysregulation of Rorgt + Foxp3 + Treg cells in Il17a Cre Il10 Flox/Flox . These cells are indeed known to be able to specifically regulate T H 17 cells, especially in the colon [34] . However, only a small fraction of Il17a Cre -activated cells are Foxp3 + and the large majority of Rorgt + Foxp3 + Treg cells are known to express little to no IL-17A and thus are not mainly affected in the small intestine of the Il17a Cre Il10 Flox/Flox mice [35] , [36] . Therefore, these data suggest that a possible dysregulation of Rorgt + Foxp3 + Treg cells is not the explanation for the selective increases in the number of T H 17 cells observed in this study. T H 17 cells also play a key role in mediating host defence against bacteria [1] . Through evolution, pathogens have developed mechanisms to evade the immune system of the host. For example, it was shown in mice and humans that S . aureus , a nosocomial and potentially multi drug resistant bacteria, promotes the anti-inflammatory fate of T H 17 cells [7] , [26] . Our data add to this because they show that the T H 17 cell anti-inflammatory fate can indeed favour dissemination of the pathogens. Given that this anti-inflammatory fate has been preserved throughout evolution, we wondered what its benefit is, and at what cost it comes. Considering that S . aureus bacteria only becomes a lethal threat when it disseminates through the blood stream, we propose that the benefit is the T H 17 cell anti-inflammatory fate’s ability to constantly maintain the immune homeostasis. We also propose that the cost of the T H 17 cell anti-inflammatory fate is rather low, considering that occurrence of a bacterial infection through the blood is relatively unlikely. The role of TGF-β during the differentiation of T H 17 cells has been widely studied and also debated [9] , [37] . It is currently accepted that TGF-β is sufficient, but not necessary for the induction of these cells and in addition, that it favours the development of T H 17 with regulatory potential. Our experiments aimed to expand the understanding of TGF-β function from the early differentiation phase to the effector phase of T H 17 cell biology. We showed for the first time directly in vivo that Tgfbr2 -deficient T H 17 cells had an impaired capacity to produce IL-10. In addition, the Tgfbr2 Flox/Flox Fate + mice phenocopied the impairment in immune regulation observed in the Il17a Cre Il10 Flox/Flox mice. These results broaden the state of knowledge of TGF-β, revealing the role of TGF-β in plasticity and function of T H 17 cells upon maturation. Furthermore, we noticed that under steady state conditions and after anti-CD3 mAb treatment, the frequency of YFP + cells increase when TGF-βRII signalling is impaired. This suggests that the expansion of T H 17 cells, which could otherwise lead to pathogenicity, is controlled by TGF-β. This is in line with the known anti-proliferative effect of TGF-β on CD4 + T cells [38] . Furthermore, we observed that the large majority of TGF-βRII deficient YFP + cells lose the expression of IL-17A under steady state conditions and upon transfer into Rag1 −/− mice, while they maintain the expression of IL-17A during intestinal inflammation. On the one hand, this is in keeping with the concept of a “sufficient but not necessary” role of TGF-β during the differentiation of T H 17 cells: under certain conditions, TGF-β is necessary to maintain IL-17A expression, but during inflammation it becomes unnecessary. On the other hand, this also suggests that the fraction of T H 17 cells which do lose IL-17A, but express IL-10 in wild type mice during inflammation have restrained the TGF-β signalling towards Smad3/ Il10 thus avoiding the re-activation of RORγt/IL-17A pathway. It has indeed been shown that TGF-β blocks RORγt activity via Smad3 [19] and that TGF-β can restrain IL-17A by a post-translational deubiquitination of RORγt [28] . Of note, TGF-β appears to impact IL-10 production also in other effector CD4 + T cells such as T H 1 cells, although the current evidence is controversial. For example, TGF-β has been shown to inhibit IL-10 production in T H 1 cells by blocking the expression of Blimp-1 [39] , while others reported a positive effect of TGF-β on IL-10 production by T H 1 cells [40] , [41] . Therefore, TGF-β seems to have different effects on T H 1 and T H 17 cells regarding IL-10 production, but further in vivo studies on T H 1 cells are required to confirm this. Downstream of TGF-β receptor, our results suggest that the canonical TGF-β mediators Smad3 and Smad4—but not TIF1-γ—promote the expression of IL-10 in mature T H 17 cells. Apparently in contrast to our data, it has been shown that TIF1-γ blocks the expression of IL-10 in CD4 + T cells while differentiating into T H 17 cells [22] . However, while this study used the CD4 Cre Tif1g Flox / Flox mouse model, we used an Il17A Cre Tif1g Flox / Flox mouse model instead. One possible explanation is that during T H 17 cell differentiation, TIF1-γ constrains IL-10 expression by obstructing Smad-recognized cis -elements from the Smad4-Smad2/3 complexes, and that this becomes dispensable in mature T H 17 cells when the Il10 gene is already accessible. In keeping with the different function of TIF1-γ in the two different phases, this is also evident regarding the regulation of IL-17A expression: TIF1-γ plays a key role in the expression of IL-17A during T H 17 cell differentiation [22] . However, our data suggest that its deletion in mature T H 17 cells becomes dispensable for IL-17A expression. Therefore, these datasets are -probably- not incompatible with each other, but rather they reveal different molecular mechanisms operating during the differentiation and maturation phases of T H 17 cells. Cell clones of blood derived human T H 17 cells are capable of acquiring the expression of IL-10 in vitro [26] . In line with this data, here we show that human primary T H 17 cells are also able to produce IL-10 and are present in the human intestine. It has recently been suggested that IL-27 promotes the expression of IL-10, via the transcription factor c-Maf, in human T H 17 clones [16] . However, whether IL-27 alone or in combination with TGF-β can also induce the expression of IL-10 in freshly isolated human T H 17 cells remains to be tested. Nevertheless, our data serve as proof of principle to show that it is possible to turn freshly isolated human T H 17 cells into IL-10 producer cells. The transcription factor Blimp1 has also been proposed as being able to promote the conversion of T H 17 cells into T R 1 cells [14] . However, it is also known that TGF-β blocks Blimp1 activation [39] , [42] . Because of this, we did not investigate the role of Blimp1 in our system. However, our data do not exclude a role of Blimp1 in the anti-inflammatory fate of T H 17 cells and it could be possible that TGF-β and IL-27 are two complementary pathways to induce the conversion of T H 17 cells into T R 1 cells in different microenvironments. Collectively, our data show that the anti-inflammatory fate of T H 17 cells is not a mere consequence of immune homeostasis, but that it actually plays an indispensable role in the maintenance of this equilibrium. TGF-β mediates the expression of IL-10 via Smad3 and Smad4 and consequently, it is the fundamental environmental signal to tighten the balance between the pro- and anti-inflammatory fates of mature T H 17 cells. We propose that the T H 17 cell plasticity between pro and anti-inflammatory fates is a key feature of immune system adaptation and when impaired, immunity and tissue integrity are compromised. Exploring the molecular mechanisms of this biological phenomena will help to identify therapeutic targets, such as Smad3 and Smad4 for new therapies that aim to steer the immune response according to the clinical need, rather than globally suppress it, as the majority of the current therapies have been based upon. Mice C57BL/6 Rag1 −/− mice (Stock #: 002216) and Rosa26 - Cas9 knock-in mice (Stock #: 028555) were purchased from the Jackson Laboratories. Il10 Flox / Flox mice (kindly provided by Axel Roers) were further crossed with Il17A Cre mice (kindly provided by Dr. Brigitta Stockinger). Tgfbr2 Flox / Flox (purchased from JAX, Stock #: 012603), Smad4 Flox / Flox (kindly provided Dr. Elizabeth Robertson [43] ) and Tif1g Flox / Flox (kindly provided by Dr. Vesa Kaartinen [44] ) mice were further crossed with Fate + mice ( Foxp3 RFP , Il10 eGFP , Il17A CRE / Katushka , R26 YFP , as described before [7] ) to generate Tgfbr2 Flox / Flox Fate + ( Tgfbr2 Flox / Flox , Foxp3 RFP , Il10 eGFP , Il17A CRE / Katushka , R26 YFP ), Smad4 Flox / Flox Fate + ( Smad4 Flox / Flox , Foxp3 RFP , Il10 eGFP , Il17A CRE / Katushka , R26 YFP ) and Tif1g Flox / Flox Fate + ( Tif1g Flox / Flox , Foxp3 RFP , Il10 eGFP , Il17A CRE / Katushka , R26 YFP ) mice. In these models, cells expressing a high level of Il17a activate the CRE recombinase to delete the stop sequence 5′ to YFP and to deplete Tgfbr2 , Smad4 or Tif1g . Thus, such IL-17A-expressing cells are permanently marked by YFP and in the meantime, lose the expression of Tgfbr2 , Smad4 or Tif1g genes. All mice were kept under specific pathogen-free (SPF) conditions, on a 12/12 on/off light cycle, maintained at 72 (+/−2) °F with 70% humidity in the animal facility at Yale University. Age- and sex-matched littermates between 8 to 24 weeks of age were used for experiments. Unless they came with special instructions, mice were randomly assigned to different experimental groups and each cage contained animals of all different experimental groups. Both male and female mice were used in experiments. Animal procedures were approved by the Institutional Animal Care and Use Committee (IACUC) of Yale University. Preliminary experiments were tested to determine sample sizes, taking available recourses and ethical use into account. Anti-CD3 mAb treatment and intestinal histology Anti-CD3 mAb (Clone #: 2C11) were injected intra-peritoneally three times (15, 15, and 30 μg per mouse) every other day. Mice were euthanised with CO 2 24 h after the last injection. Different parts of small intestines (duodenum, jejunum and ileum) were fixed in Bouin’s Fixative Solutions for 1 h. Tissues were then embedded in paraffin for sectioning. Pictures were taken by optical microscope equipped with camera systems and analysed. Lymphocyte isolation from mouse small intestine Methods were described before in detail [45] . Basically, intestinal tissues were first digested in 1 mM DTE at 37 °C for 30 min to get the IEL fraction. Remaining tissues were then digested in 1 mg/ml collagenase from Clostridium Histolyticum at 37 °C for another 30 min to get the LPL fraction. Both fractions were further applied with Percol gradient centrifugation to enrich lymphocyte populations. Flow cytometry antibodies and intracellular cytokine staining Mouse T cells were stained with monoclonal antibodies to CD4 (GK1.5, Cat # 100428 or RM4-5 Cat # 100536), CD8 (53-6.7 Cat # 100722), NK1.1 (PK136 Cat # 108713), CD19 (6D5 Cat # 115508), CD11b (M1/70 Cat # 101216), CD11c (N418 Cat # 117318), γδTCR (GL3 Cat # 118123), TGFβRII (R&D Systems Cat # FAB532P). All antibodies without further instructions are purchased from eBiolegend and diluted 1:200 for staining at 4 °C. Importantly, TGFβRII staining was performed at 37 °C for 30 min with 1:50 dilution. 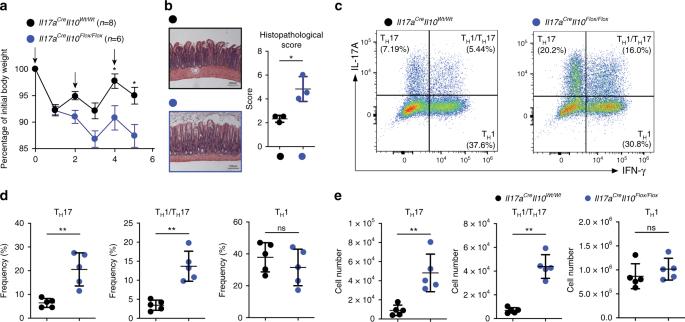Fig. 3: IL-10 deletion in TH17 impairs intestinal immune regulation. aPercentage of initial body weight after anti-CD3 mAb. The arrows indicate the injection of anti-CD3 mAb. Data are cumulative of three independent experiments. Mean ± SEM.; *P< 0.05, by two-way ANOVA with Bonferroni’s post test.bRepresentative histological pictures of H&E stained small intestines after anti-CD3 mAb treatment. For the statistical analysis on the right, one representative experiment out of two is shown. Each dot represents one mouse (nwild type= 3,nKO= 3). Mean ± S.D.; *P< 0.05 by Welch’st-test.cFlow cytometric analysis of small intestinal CD4+T cells after anti-CD3 mAb treatment. Small intestinal lymphocytes were isolated from the indicated mouse lines and intracellular staining for both IL-17A and IFN-γ was performed to identify TH17 (IL-17A+IFN-γ−), TH1/TH17 (IL-17A+IFN-γ+) and TH1 (IL-17A−IFN-γ+) cells. A pre-gate on CD4+cell is applied.d,eStatistical analysis of frequencies (d) and numbers (e) are shown. One representative experiment out of three is shown. Each dot represents one mouse (nwild type= 5,nKO= 5). Mean ± S.D.; ns, not significant; **P< 0.01 by Mann–WhitneyUtest. Source data are provided as a Sourcedatafile. Although in the figure legends we referred only to CD4 + T cells, in each FACS related experiment we specifically analysed CD4 + T cells CD8 − , NK1.1 − , CD19 − , CD11b − , CD11c − , γδTCR − . For intracellular cytokine staining, the cells were re-stimulated for 3 h at 37 °C with phorbol 12-myristate 13-acetate (PMA) (Sigma, 50 ng ml −1 ) and ionomycin (Sigma, 1 μg ml −1 ) in the presence of Golgistop (BD Bioscience). Cells were then fixed in 3.7% formaldehyde for 20 min at room temperature. After washing, the cells were then permeabilized in 0.1% NP40 and stained at 37 °C with anti-IL-17A (TC11-18H10.1 Cat # 506925), anti-IFNγ (BD Bioscience, Cat # 554412) antibodies for 30 min with 1:200 dilution. Lymphocytes were re-suspended in PBS, 0.5% FBS, 5 mM EDTA and acquired with an LSRII cytometer (BD Bioscience). Staphylococcus aureus infections Heat-inactivated S. aureus (ATCC 14458, SEB+ TSST-1-) was injected intravenously (1 × 10 7 colony forming units per mouse) into 4-week-old mice for immunization purposes. Three weeks later, the mice were injected intravenously again with 1 × 10 6 live S. aureus bacteria. Mice were euthanised with CO 2 1 week after the 2nd injection, when they displayed clinical symptoms of sepsis. Different organs were then harvested to examine the colony forming unit (CFU) of S. aureus . T cells isolated from intestines were further analyzed by FACS. Plasmids and transfections The coding sequences for Smad3 and Smad4 were cloned via reverse transcription and PCR from murine C57BL/6 splenic leukocytes total RNA with the appropriate primers, Superscript III reverse transcriptase ( Invitrogen ) and Phusion® Hot Start Flex DNA polymerase ( New England Biolabs ). The PCR products were cloned in pGEM®-T Easy vector (Promega) and were subsequently sub-cloned into pCMVT N T™ (Promega) and pCMV-Tag2 (Agilent Technologies) mammalian expression vectors respectively, using the appropriate primers and the InFusion ligation system (Takara). The Il10 proximal promoter (from −1444 to +1 bp) was cloned via PCR from C57BL/6 genomic DNA with appropriate primers and was subcloned into pGL2 vector (Clontech) using the InFusion ligation system (Takara) and appropriate primer sets. Transfections were performed in HEK293T cells with the BES buffered saline/CaCl 2 method. Briefly, expression and reporter plasmid mixes were left to precipitate for 20 min at room temperature, in a solution containing 0.125 M CaCl 2 , 0.025 M BES, 0.02 NaCl, 0.00075 NaH 2 PO 4 , pH:6.95. The precipitated plasmid mix was overlaid carefully on the HEK293T cell DMEM 10% FBS culture medium. 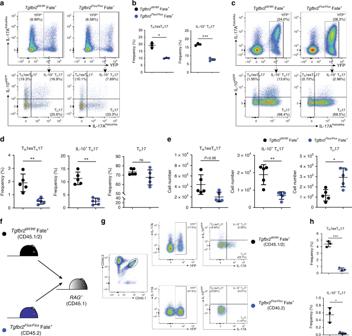Fig. 4: TGF-βRII is required for mature TH17 cells to produce IL-10. aFlow cytometric analysis of in vitro cultured total CD4+T cells. Cells were polarized under TH17 condition for 5 days. A pre-gate on viable (DAPI−), CD4+T cell population is applied.bStatistical analysis of IL-10+TH17 and TR1exTH17cells is shown by one representative experiment out of three. Each dot represents one mouse (nwild type= 3,nKO= 5). Mean ± S.D.; *P< 0.05, ***P< 0.001 by Welch’st-test.cFlow cytometric analysis of small intestinal CD4+T cells after anti-CD3 mAb treatment. The indicated reporter mouse lines were used. Top panels are pre-gated on Foxp3−CD4+T cells. Bottom panels are gated on YFP+cells, as shown, and the indicated populations are identified on the basis of the reporter molecules as follows: TR1exTH17cells: IL-10eGFP+IL-17aKata−; IL-10+TH17 cells: IL-10eGFP+IL-17aKata+; TH17 cells: IL-10eGFP–IL-17aKata+.d,eFrequencies (d) and numbers (e) of the indicated populations are shown. One representative experiment out of three is shown. Each dot represents one mouse (nwild type= 5,nKO= 5). Mean ± S.D.; ns, not significant; *P< 0.05, **P< 0.01 by Mann–Whitney U test.f. Experimental design for Co-transfer of total CD4+T cells isolated from wild-type Fate+mouse andTgfbr2Flox/FloxFate+mouse lines.g. Flow cytometric analysis of small intestinal co-transferred CD4+T cells after anti-CD3 mAb treatment. Small intestinal lymphocytes were isolated from the indicated mouse lines and intracellular staining was then performed to identify the indicated cell populations in combination with reporter molecules for IL-10 (eGFP) and IL-17a lineage (YFP). All cell populations are pre-gated on CD4+T cells.hFrequencies of TR1exTH17and IL-10+TH17 in G is shown by one representative experiment out of two. Each dot represents one recipient mouse (n= 3). Mean ± S.D.; *P< 0.05, ***P< 0.001 by Welch’st-test. Source data are provided as a Sourcedatafile. In all, 24 h later the transfection medium was aspirated and fresh DMEM 10% FBS was placed onto the HEK293T cells. Cells were collected 48 h after transfection, washed twice with PBS and lysed in Passive Lysis Buffer (Promega). Luciferase activity was determined using the Luciferase Assay System (Promega) and was measured in a FluoStar Omega reader and Software. Transfection efficiency was determined by spiking all transfections with 0.5 ng pCMV-EGFP vector (Clontech) and measuring GFP activity in the lysates. T H 17 cell differentiation and immunoblot Briefly, naïve CD4 + T cells were isolated from the spleen and lymph nodes of 4–6 mice of the indicated transgenic mouse strains with the mouse naïve CD4 + T cell isolation Kit (Stemcell). The cells were cultured for five days under T H 17 polarizing conditions, in Click’s medium supplemented with 5% FBS, 0,1 mM β-merkaptoethanol, Glutamax™ (Gibco), 100 U/mL Penicillin/Streptomycin, 10 μg/mL anti-CD3, 2 μg/mL anti-CD28, 10 μg/mL anti-IFNγ, 10 μg/mL anti-IL-4, 20 ng/mL murine IL-23, 20 ng/mL murine IL-6, 0.5 ng/mL murine TGF-β1 (unless specially indicated). T H 17 cells were sorted based on the IL-17A reporter expression resuspended into 2 × 10 6 cells/mL and then challenged with or without TGF-β for 30′ min. Subsequently the cells were lysed and either total or nuclear extracts were obtained and loaded on 4–15% precast acrylamide gels (Mini-PROTEAN, BIO-RAD). After electrophoresis the proteins were transferred to PVDF membranes. The membranes were immunoblotted with the indicated antibodies and developed according to standard protocols. We loaded the protein extract equivalent corresponding to 8 × 10 5 T H 17 cells in each well. Retroviral preparation and transduction For retroviral preparation, 1 μg of individual Smad3 sgRNA vector with 0.5 μg of EcoHelp plasmid were employed to transfect HEK293T cells. In all, 12 h later, media was replaced and virus was grown for another 48 h. Supernatant containing virus was collected and polybrene was added to achieve a final concentration of 4 μg/ml. For retroviral transduction, Cas9-expressing T cells were first activated for 24 h and then spin transduced with viral supernatant. Chromatin Immunoprecipitation Rested T H 17 cells were challenged or not with 1 μg/mL TGF-β1 for 30 min. The cells were fixed with 1.1% Formaldehyde for 10 min, washed, and re-suspended in 10 mM Tris pH:7.5, 10 mM NaCl, 3 mM MgCl 2 , 1 mM CaCl 2 , 4% NP40 supplemented with protease inhibitors, at a final concentration of 4 × 10 7 cells/mL. Subsequently, 0.2 units MNase (Sigma) were added for 5 min at 37 °C, followed by 3 mM EGTA and the cells were centrifuged at 500 g and re-suspended in 50 mM Hepes pH:7.9, 150 mM NaCl, 5 mM EDTA, 0.5 mM EGTA, 0.1%SDS, 0.1% Na-deoxycholate, supplemented with protease inhibitors and sonicated 3 times for 20 sec. 1% Triton X-100 was added and the samples were centrifuged for 15000 g for 15 min at 4 °C. The lysates were extensively dialysed in 10 mM Tris pH: 7.5, 5% glycerol, 1 mM EDTA, 0.5 mM EGTA. For immunoprecipitation, T H 17 cell lysates were incubated o/n with designated antibodies and the next day were mixed with Dynabeads™ Protein G (Invitrogen, #00374128) in RIPA buffer for 4 h at 4 °C. The beads were washed in low (150 mM NaCl), high (500 mM NaCl) and LiCl (250 mM) salt buffer, the crosslinks were reversed at 65 °C, the samples were purified by Phenol/Chlorophorm extraction, the DNA was precipitated and used in q-PCR reactions. Real-time quantitative PCR qPCR was performed using chromatin immunoprecipitation reactions with the anti-Smad3 and Smad4 and isotype control antibodies, along with the indicated primers and KAPA SYBR FAST qPCR Kit (Kapa Biosystems, Wilmington, MA) in a StepOne cycler (Applied Biosystems, Carlsbad, CA). 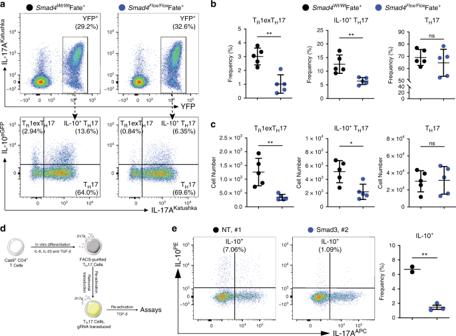Fig. 5: TGF-β signals via Smad3/4 to regulate IL-10 in TH17 cells. aFlow cytometric analysis of small intestinal CD4+T cells after anti-CD3 mAb. The indicated reporter mouse lines were used. Top panels are pre-gated on Foxp3−, CD4+T cells. Bottom panels are pre-gated on YFP+cells, and the indicated populations are identified on the basis of the reporter molecules as follows: TR1exTH17cells: IL-10eGFP+IL-17aKata−; IL-10+TH17 cells: IL-10eGFP+IL-17aKata+; TH17 cells: IL-10eGFP−IL-17aKata+.b,cFrequencies (b) and numbers (c) of TR1exTH17, IL-10+TH17 and TH17 cells in A are one representative experiment out of three. Each dot represents one mouse (nwild type= 5,nKO= 5). Mean ± S.D.; ns, not significant; *P< 0.05, **P< 0.01 by Mann-–WhitneyUtest.dExperimental design of knocking out Smad3 in in vitro differentiated mature TH17 cells by using CRISPR/Cas9 technology.eFlow cytometric analysis of in vitro cultured mature TH17 cells after knocking out Smad3 by using gRNAs targeting Smad3. Cells were pre-gated on viable CD4+T cells. NT, non-targeting control. Each dot represents an individual gRNA (nNT= 2,nSmad3= 3). Mean ± S.D.; **P< 0.01 by Welch’st-test. Source data are provided as a Sourcedatafile. The CT values from triplicate qPCR reactions were extracted from the StepOne cycler (Applied Biosystems, Carlsbad, CA) onto spreadsheets and were analyzed with the relative quantification method 2 –ΔΔCT . The abundance level of a given amplicon per sample/condition was determined relative to its input (non-enriched) chromatin abundance and was additionally corrected relative to isotype control antibody immunoprecipitation sample. Proximity ligation assay In vitro differentiated sorted T H 17 cells were rested for 5 days in Click’s medium supplemented with 2 ng/mL murine IL-2 (PeproTech #212-12) and were subsequently challenged with 1 μg/mL human TGF-β1 for 30 min. Subsequently, the cells were washed, re-suspended in a minimal volume of PBS supplemented with 10% FBS 0.3% BSA, overlaid onto coverslips and were left to dry for 12 h. The cells were rehydrated with PBS, fixed with 4%PFA and permeabilized with 0.3% PBS-Triton X100. After washing, the specimens were blocked, incubated with pospho-Smad3 and Smad4 antibodies and stained with Duolink® In Situ detection Reagents Red (Sigma). After mounting, the slides were analysed by confocal microscopy and the acquired images were opened and processed with Fiji software (Image J). Lymphocyte isolation from human intestine The human colonic tissue is derived from colon cancer patients admitted into the UKE General Surgery Clinic. The study was approved by the Ethical Physicians Committee of Hamburg (Ethik-Kommision der Aertztekammer Hamburg) and Informed Written Consent was obtained from each one of the sample donors. The general characteristics of the participants cohort were five males and nine females with an average age of 69,5 years (±SD = 11 y ) Healthy tissues adjacent to the tumor, were collected by collaborating surgical personnel, immediately after the completion of the surgical procedure. Next, the tissue samples were processed for lymphocyte isolation. Intraepithelial lymphocytes were isolated by digesting the tissue with Dithiothreitol (DTT Sigma-Aldrich) solution at 37 °C for 20 min, followed by incubation with collagenase IV (100 U; Sigma-Aldrich) for 30 min at 37 °C. The cells were further separated by a Percoll gradient (GE Healthcare). After this the cells were stained for FACS analysis. Only the healthy colonic tissue data analysis with respect to CD4 + FOXP3 − IL17A + and IL-10 + cell compartment is presented in this manuscript. For a comprehensive description of the patients, please refer to the Source data file of Supplementary Fig. 9e . Part of the human cohort analyzed in this study was also used for assessing the expression of IL-22 in Perez et al. [46] . Sorting of humanT H 17 cells from Buffy Coat Enriched human Buffy Coat samples retrieved directly from the UKE Transfusion Medicine, were diluted with PBS to a total volume of 350 mL. The diluted blood samples were overlaid to buffered Biocoll separating solution (Merck, #L6715) and centrifuged at 300 g for 20 min. The PBMCs were collected, washed with PBS and stimulated for 3 h with 50 ng/mL PMA and 1μΜ Ionomycin. CD4 + T cells were selected with magnetic human CD4 microbeads (#130-045-101, Miltenyi, Bergisch-Gladbach, Germany). IL-17 + cells were stained with the IL17A secretion assay detection kit (#130-094-537, Miltenyi, Bergisch-Gladbach Germany) and with human anti-CD4/FITC, anti-CD45RA/Alexa700, anti-CD127/PE.Cy7 and anti-CD25/BV650 and sorted with an Aria Illusion instrument (BD Bioscience). In all, 5–8 × 10 3 sorted CD4 + IL-17A + CD45RA − CD127 − CD25 − cells were rested in RPMI medium (supplemented with 10% FBS, 10 mM β-merkaptoethanol, Glutamax, Penicillin/Streptomycin 100 U/mL) plus 2 ng/mL IL-2 (PeproTech). After 48 h the cells were challenged with increasing concentrations of TGF-β1 for five days. Subsequently, cells were stimulated with PMA/Ionomycin, stained for CD4, IL-17A, and IL-10 expression and analysed by FACS. Statistics FACS data were visualized and analyzed with FlowJo 10.5.3 (BD Bioscience). Statistical analyses were calculated in Prism (Graphpad Software). According to the experimental set-up we used Mann–Whitney U test or Welch’s t -test (Data specified in Figs. 1 – 5 ), two-way ANOVA (Fig. 6b ) and χ 2 test (Fig. 6d ). The p values presented in Fig. 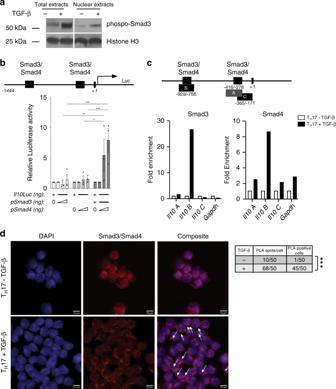Fig. 6: Smad3 and Smad4 activateIl10transcription in TH17 cells. aWestern blot of TH17 cell-total/nuclear extracts challenged with or without TGF-β for 30 min. One representative experiment out of two is shown.bSchematic representation of the proximal murineIl10promoter (from −1444 to +1 bp) driving the expression of the luciferase reporter gene (luc). The predicted binding sites for Smad3 and Smad4 as well as theIl10TSS are depicted (top). Relative Luc activity driven by Smad3 and Smad4 on proximalIl10promoter (bottom). Mean ± SEM (n= 3). *P< 0.05, **P< 0.01, and ***P< 0.001 by ordinary two-way ANOVA and Tukey’s multiple comparisons test.cSchematic representation of the proximal murineIl10promoter (from −1444 to +1 bp) indicating the predicted binding sites for Smad3 and Smad4 and the depicted amplicons A (from −416 to −278 bp), B (from −929 to −756 bp), and C (from −365 to −171 bp) (top) that were used to amplify the chromatin Immunoprecipitated DNA. Smad3 and Smad4 Chromatin immunoprecipitation (ChIP) of sorted TH17 cells challenged with or without TGF-β (bottom). One representative experiment out of three is shown.dProximity Ligation Assay (PLA) using sorted TH17 cells challenged with or without TGF-β. White arrows indicate positive Smad3/Smad4 interaction signal (red dots) superimposed on nuclei stained with DAPI (blue). Scale bar represents 10 μm. Number of PLA spots per cell and the number of PLA positive cells are reported in the box. One representative experiment out of two is shown. ***P< 0.001 for comparison byχ2test. Source data are provided as a Source datafile. 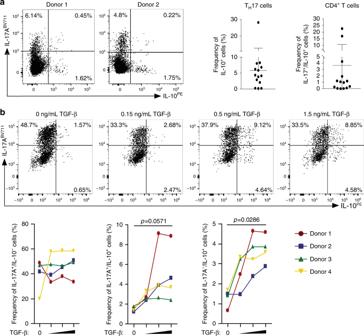Fig. 7: TGF-β promotes IL-10 expression in human TH17 cells. aTwo representative dot plots of CD4+T cells extracted from healthy human colonic tissue, stained intracellularly for IL-17A and IL-10. The diagrams show the frequencies of IL-17A+/IL-10+within the TH17 cells (left) and within the total CD4+T cell (right) (n= 14)bRepresentative dot plots of TH17 cells isolated from human blood donor, stimulated and cultured under increasing TGF-β1 concentrations for 5 days and finally stained for IL-17A and IL-10 intracellularly. The graphs below show the percentages of IL-17A+/IL-10−, IL-17A+/IL-10+and IL-17A−/IL-10+cells from four different blood donors.Pvalues were calculated between the lowest TGF-β and highest TGF-β concentration conditions by Mann–WhitneyUtest (n= 4). Source data are provided as a Source data file. 7 were calculated via the Mann–Whitney U test. The specific statistical analyses used in each figure are further described in the figure legends. When not otherwise specified, the statistical test used is always two-sided. p < 0.05 was considered significant. Reporting summary Further information on research design is available in the Nature Research Reporting Summary linked to this article.